Uncovering loss mechanisms in silver nanoparticle-blended plasmonic organic solar cells There has been much controversy over the incorporation of organic-ligand-encapsulated plasmonic nanoparticles in the active layer of bulk heterojunction organic solar cells, where both enhancement and detraction in performance have been reported. Here through comprehensive transient optical spectroscopy and electrical characterization, we demonstrate evidence of traps responsible for performance degradation in plasmonic organic solar cells fabricated with oleylamine-capped silver nanoparticles blended in the poly (3-hexylthiophene):[6,6]-phenyl-C 61-butyric acid methyl ester active layer. Despite an initial increase in exciton generation promoted by the presence of silver nanoparticles, transient absorption spectroscopy reveals no increase in the later free polaron population—attributed to fast trapping of polarons by nearby nanoparticles. The increased trap-assisted recombination is also reconfirmed by light intensity-dependent electrical measurements. These new insights into the photophysics and charge dynamics of plasmonic organic solar cells would resolve the existing controversy and provide clear guidelines for device design and fabrication. Bulk heterojunction (BHJ) organic solar cells (OSCs) comprising of bi-continuous networks of a semiconducting polymer/fullerene derivative have been under intense scrutiny in the recent years because of their attractive properties such as light weight, high flexibility, cost effectiveness, ease of fabrication, and so on. The power conversion efficiencies (PCEs) of such cells have attained the 8−10% mark [1] , [2] . One of the main bottlenecks in improving efficiencies is ascribed to the trade-off between light absorption and charge extraction, which restricts the active layer thickness. Light-trapping strategies utilizing plasmonic metallic nanostructures as light concentrators offer a highly attractive solution to this predicament. For instance, metallic nanoparticles (NPs) have been commonly employed as subwavelength antennas and scattering centres to enhance the absorption of BHJ films [3] . Typically, these metal NPs are either embedded in the charge transfer layer such as PEDOT:PSS [4] , [5] , [6] , [7] or simply blended within the active BHJ layer [8] , [9] , [10] , [11] . In the latter approach, NPs coated with organic ligands are typically used to disperse the particles within the organic blends. Despite its simplicity, the findings from this approach are highly controversial as both enhancement [8] , [9] , [10] , [11] and detraction [12] , [13] in organic photovoltaic (OPV) devices performance have been reported. Physical insight into the fundamental photophysics and charge dynamics in these NP-blended plasmonic OPV cells is urgently required. Investigating the fundamental photophysical and dynamical processes governing charge generation, recombination and extraction in these hybrid plasmonic films, and correlating them to the electrical properties/device performance of functional devices are the main foci of this work. Here, we present a comprehensive transient optical spectroscopy and electrical characterization study of the carrier dynamics and transport in thin films and devices fabricated using a representative hybrid plasmonic OPV system comprising of oleylamine-capped silver nanoparticles (AgNPs) blended within poly (3-hexylthiophene):[6,6]-phenyl-C 61-butyric acid methyl ester (P3HT:PCBM) films. Transient optical studies spanning the temporal regimes of charge generation, recombination, transport and extraction (that is, over 7 orders of magnitude from 100 fs to 5 μs) were used to probe the system. Femtosecond transient absorption spectroscopy (fs-TAS) revealed that while the initial exciton generation density improved with the incorporation of AgNPs, there is also a higher rate of polaron quenching in the AgNPs-P3HT:PCBM blends compared with the P3HT:PCBM control blends—ascribed to the fast trapping of polarons by the AgNPs. Nanosecond transient absorption spectroscopy (ns-TAS) uncovered the presence of fast trap-assisted recombination—attributed to increased subgap trapping states at the interfacial region of P3HT:PCBM originating from the AgNPs. Intensity-dependent open-circuit voltage ( V OC ) and dark current measurements confirmed the increased trap density (that is, increased disorder in the density of states) that leads to higher trap-assisted recombination. Our findings provide new insights into the fundamental photophysics and charge dynamics in plasmonic OSCs. Importantly, our work sheds light on the present controversy regarding the positive and negative influence of adding AgNPs to the BHJ. On the basis of these findings, we have also provided suggestions and guidelines for developing high-performance hybrid plasmonic OSC devices. Fabrication and physical characterization Fabrication of AgNPs using oleylamine as both surfactant and reducing agent is a simple, inexpensive, versatile and highly reproducible method. The size of the metallic NPs could be easily tuned using the reaction temperature and larger particle sizes for better light scattering could be achieved [14] . The as-synthesized AgNPs had an average diameter of ~24.7 nm (measured through transmission electron microscopy, see Supplementary Fig. S1 inset). Steady-state optical absorption spectra of AgNPs in 1,2-dichlorobenzene (DCB) indicated a peak at 417 nm, corresponding to localized surface plasmon resonance peak of the AgNPs in DCB ( Supplementary Fig. S1 ). A comparison of the optical absorption in the bare P3HT:PCBM control film and the AgNPs-P3HT:PCBM films indicated an enhanced absorption over a broad region for the AgNP-embedded film, which can be ascribed to be plasmonic in origin (that is, enhanced local electromagnetic field and strong far-field scattering) [3] , [15] . Furthermore, the three vibronic peaks/shoulders of P3HT (at ~510 , ~560 and ~600 nm, corresponding to the 0–2, 0–1 and 0–0 vibronic transitions of P3HT) do not exhibit any prominent shift or relative magnitude variation with increasing volume ratios of AgNPs in the BHJ films, indicating that the crystalline order of P3HT is not significantly compromised [16] . Charge dynamics in the fs-ns temporal regime Transient absorption were performed on 100-nm-thick P3HT:PCBM control films and AgNPs-P3HT:PCBM films. 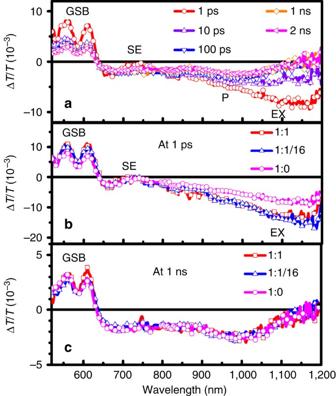Figure 1: The effect of AgNPs on the exciton and polaron generation observed via fs-TAS. (a) Relative differential transmission (ΔT/T) of P3HT:PCBM ranged from 520 nm to 1,200 nm. Selected times are 1 ps, 10 ps, 100 ps, 1 ns and 2 ns after excitation with 500-nm laser beam. A comparison of the fs-TAS signals of Ag-P3HT:PCBM and P3HT:PCBM BHJ films at (b) 1 ps and (c) 1 ns after photoexcitation. Figure 1a shows the representative differential transmission (DT) spectra spanning 520–1,200 nm for the control samples at different delay times following photoexcitation. The vibronic peaks corresponding to 0–0 and 0–1 absorption transitions (520–620 nm) manifest as ground state bleaching (GSB) peaks [16] . This photobleaching signal (that is, Δ T / T >0 or relative DT>0), which arises from the state-filling of the excitonic and polaronic states, is proportional to the population of the excitons and polarons in the photoexcited films [17] . The negative Δ T / T signal centred at ~700 nm is attributed to the photo-induced absorption (PIA) of photogenerated delocalized polarons in the crystalline P3HT domains. The spectrum at 1 ps shows a weak positive peak around 740 nm (within the broad negative PIA band) that arises from the stimulated emission of P3HT singlet excitons [16] , [18] . This peak disappears within 10 ps due to the fast quenching of P3HT excitons by the PCBM acceptor. In the near-infared region (NIR), there is a broad PIA peak centred around 1,150 nm at 1 ps, which subsequently decays within 100 ps. Following which, a long-lived (ns) PIA peak centred around 1,000 nm remains. The PIA peak at 1,150 nm is ascribed to singlet excitons (EX) while the 1,000 nm peak originates from an overlap of signals from P3HT singlet excitons, P3HT polarons (P) in disordered domains and PCBM anions [17] , [18] . At 1-ps delay, the PIA peak at 1,150 nm originates from the singlet exciton population present in the films, while at 1-ns delay the PIA peak at 1,000 nm originates predominantly from the polaron population present. Monitoring the relative magnitudes of these DT signals at 1,150 nm and 1,000 nm allows us to compare the relative populations of the residual excited species at the respective times following photoexcitation and evaluate the effect of AgNPs on the charge generation and recombination. Figure 1: The effect of AgNPs on the exciton and polaron generation observed via fs-TAS. ( a ) Relative differential transmission (Δ T / T ) of P3HT:PCBM ranged from 520 nm to 1,200 nm. Selected times are 1 ps, 10 ps, 100 ps, 1 ns and 2 ns after excitation with 500-nm laser beam. A comparison of the fs-TAS signals of Ag-P3HT:PCBM and P3HT:PCBM BHJ films at ( b ) 1 ps and ( c ) 1 ns after photoexcitation. Full size image Figure 1b shows the DT signals at 1-ps delay for the control and two AgNPs-P3HT:PCBM samples (that is, with low (1:1/16) and high (1:1) AgNPs concentrations plotted for clarity). The absolute magnitudes at 1,150 nm are more pronounced in the AgNPs-P3HT:PCBM blends compared with the control with an estimated increase of ~27 and 31% (over the 0–1 ps timescale, not shown in the report) for the low and high AgNPs concentrations, respectively. This indicates that the rate of singlet exciton generation is indeed enhanced by the presence of the AgNPs. However, at 1-ns delay ( Fig. 1c ), the magnitude of the DT signals is almost invariant in all the samples, indicating that a comparable polaron population is present in all the samples. This clearly indicates that an increase in singlet exciton population brought about by the plasmonic enhancements does not translate to a corresponding increase in the free carrier population. There are several possible mechanisms for this asymmetric behaviour: ( M1 ) a higher rate of exciton recombination stemming from an increased radiative recombination rate and/or an increased non-radiative recombination through Förster resonant energy transfer, Dexter energy transfer and exciton trapping in the presence of AgNPs; ( M2 ) the high density of excitons and charges induced by strong local field enhancement could increase the probability of bimolecular recombination through exciton–exciton, exciton–polaron, polaron–polaron annihilation, which depletes the polaron population; ( M3 ) trapping and loss of polarons at defects and impurities. The dynamics of the PIA bands would allow us to trace the evolution of the respective species and elucidate the origin of this asymmetry. 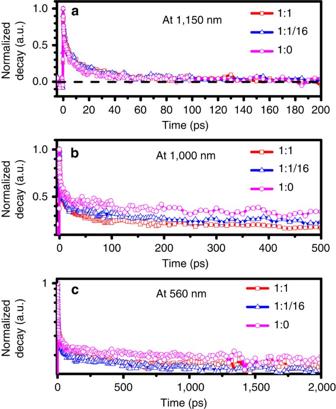Figure 2: Transient decays of AgNPs-P3HT:PCBM and P3HT:PCBM BHJ films. (a) The singlet exciton decay monitored at 1,150 nm. (b) The signal at 1,000 nm is a superposition of exciton and polaron decay. (c) GSB decay monitored at 560 nm. Figure 2a shows the decay transients of the singlet excitons (or the recovery of the PIA signals back to the equilibrium) at 1,150 nm for the control and the 1:1/16 and 1:1 ratio AgNPs-P3HT:PCBM samples. The invariance in the singlet exciton lifetimes in all the samples indicates that its recombination dynamics are not affected by the presence of the AgNPs in the blends and is therefore inconsistent with ( M1 ). Time-resolved photoluminescence (TRPL) measurements indicated the invariance of the exciton lifetime (monitored between 650 and 710 nm)—in concurrence with these TA findings—see Supplementary Fig. S2 . This is not surprising as the emission of the P3HT excitons at ~650–710 nm has minimal overlap with the localized surface plasmon resonance peak of the AgNPs, ruling out Förster resonant energy transfer [19] , while the long oleylamine ligand spacers reduce the probability of Dexter energy transfer [20] . To scrutinize the possibility of increased exciton–exciton, exciton–polaron, polaron–polaron annihilation ( M2 ), pump power-dependent measurements were performed. At high exciton/polaron densities, the unvarying exciton and polaron population at the relevant time scales [17] (see Supplementary Fig. S3 ) indicate that higher order recombination is not significant in affecting the polaron formation, thus ruling out M2 . Figure 2: Transient decays of AgNPs-P3HT:PCBM and P3HT:PCBM BHJ films. ( a ) The singlet exciton decay monitored at 1,150 nm. ( b ) The signal at 1,000 nm is a superposition of exciton and polaron decay. ( c ) GSB decay monitored at 560 nm. Full size image Figure 2b shows the normalized DT transients at 1,000 nm over a timescale of 500 ps (that is, with signals from both the P3HT singlet excitons and the free polarons). Differences in the DT transients for the control and the two AgNPs-P3HT:PCBM samples occur within 100 ps—that is, in the realm when exciton diffusion and dissociation into free polarons are completed. This indicates that the incongruence in the polaron population (with respect to the initial singlet exciton population) arises from ( M3 )—a fast trapping of the polarons by the AgNPs. Furthermore, a fraction of these trapped charges could also undergo fast recombination at the P3HT:PCBM interface, as the GSB decay transient at 560 nm shows a slight decrease in magnitude of the long-lived component (which is ascribed to the free and trapped polarons)—see Fig. 2c . Although exciton generation is increased by the presence of these oleylamine-coated AgNPs, these AgNPs could also function as traps for the polarons in its locality—thus negating any increase in the polaron population. Next, ns-TAS will allow us to monitor the dynamics of the long-lived polarons. 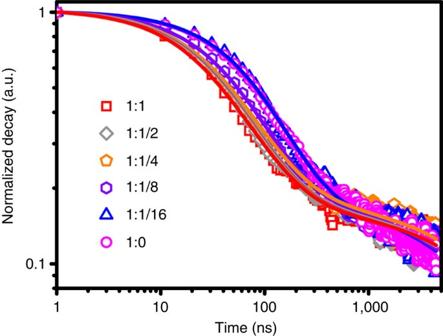Figure 3: Transient decays of AgNPs-P3HT:PCBM and P3HT:PCBM at 560 nm measured by ns-TAS. Pump wavelength was 500 nm and the fluence used was ~60 μJ cm−2. Solid lines are the fitted curves. Polaron dynamics in the ns-μs temporal regime Figure 3 shows the DT decay transients from ns-TAS at the GSB peak of 560 nm for the samples following pump excitation with ~60 μJ cm −2 fluence. A fast decay is followed by a long-lived tail extending beyond our TAS time window. We model the recombination process as comprising of both monomolecular (first order) and bimolecular (second order) processes. The bimolecular process is usually described by Langevin recombination, which occurs when two free opposite charges (originating from different excitons) recombine. On the other hand, monomolecular recombination is often reported as Shockley-Read-Hall (SRH) like trap-assisted recombination process, when one free charge recombines with another charge immobilized at an interfacial trap state [21] , [22] . As an approximation, we consider that these two processes occur independently where a fraction ( f ) of the initially generated charges undergo bimolecular recombination while the rest (1— f ) undergo monomolecular (first order) recombination [23] , [24] . To account for the measurements being performed at high fluence, we included a carrier concentration-dependent mobility μ ∝ N α —as a consequence of energetic disorder on the hopping of thermally activated charge carriers [25] , [26] , [27] , [28] , [29] , where α is the concentration-dependent exponent [23] . Hence, the expressions are: Figure 3: Transient decays of AgNPs-P3HT:PCBM and P3HT:PCBM at 560 nm measured by ns-TAS. Pump wavelength was 500 nm and the fluence used was ~60 μJ cm −2 . Solid lines are the fitted curves. Full size image where N mon and N bim refers to charges undergoing monomolecular and bimolecular recombination, respectively; γ 1 and γ 2 are the recombination prefactors; and , . k 1 and k 2 are related to the recombination rates for monomolecular and bimolecular processes, respectively. The third expression is a sum of both contributions and corresponds to the TAS signal of the GSB. This model was also successfully validated for pump fluence-dependent increase of the recombination rate (data not shown). The extracted parameters are listed in Table 1 . The concentration-dependent exponent α for P3HT:PCBM is very close to the reported values [24] . From the fits, it is clear that majority of charges undergo trap-assisted recombination in the P3HT:PCBM system (as indicated by the low value of f ). Earlier reports had concluded either a negligible [30] , [31] , or a dominant Langevin process in P3HT:PCBM [32] . This difference may be ascribed to the different models used or the different excitation fluence used, as Langevin processes dominate with increasing pump fluence because of its bimolecular characteristics. The primary difference among the AgNP-embedded cells and control cells is k 1 , which is determined by the trap density and capture coefficients. k 1 increases by three times with increased AgNP concentration while k 2 remains relatively insensitive. This indicates that the subgap trap density increases with the incorporation of AgNPs, functioning as recombination centres for photoexcited charges. The traps may originate from the metal core of the AgNPs due to ineffectual oleylamine ligand coverage. Some functional groups in the ligand may also provide localized states. Topp et al. [12] had previously shown that gold nanoparticles encapsulated with different ligands (that is, with dodecylamine, pyridine, and so on) all had detrimental effects on the PCE of P3HT:PCBM OSCs. There is still a lack of understanding on how the capping ligands and particle size affect the net trapping rate. However, it is not the focus of this study to unravel these dependencies. The presence of trap states in AgNP-embedded P3HT:PCBM films are next confirmed through electrical characterization of the photovoltaic devices. Table 1 Fitted parameters of the ns-TAS data. Full size table Photovoltaic characterization Inset of Fig.4 shows the schematic of a typcial plamsonic OSC. Following established procedures, the devices were post-annealed to improve efficiency. Typical current density–voltage ( J–V ) curves and incident photon-to-electron conversion efficiency (IPCE) of the control and the AgNPs-P3HT:PCBM devices are given in the Fig.4 and Supplementary Fig. S4 , respectively. Details of their device performance parameters are also listed in Table 2 . The control devices (with no AgNPs) yielded a PCE of 3.1%. The PCEs, fill factors (FFs) and V OC s decrease with increasing AgNPs concentration. The J SC on the other hand fluctuates, but is typically less than that of the control. The IPCE results are consistent with the J–V measurements, where the external quantum efficiency decreases with increasing AgNPs concentration. 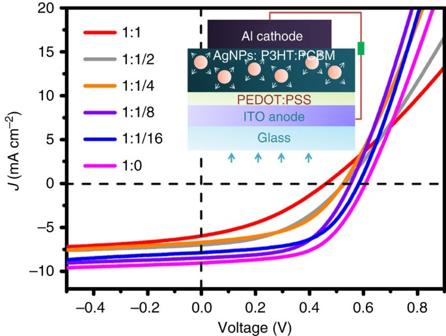Figure 4: Device performances of hybrid plasmonic OSCs. J–Vcurves of AgNPs-P3HT:PCBM and P3HT:PCBM OSCs. Figure 4: Device performances of hybrid plasmonic OSCs. J – V curves of AgNPs-P3HT:PCBM and P3HT:PCBM OSCs. Full size image Table 2 Electrical performance of post-annealed AgNPs-P3HT:PCBM and P3HT:PCBM OSCs. Full size table Intensity-dependent V OC measurements Intensity-dependent open-circuit voltage measurements were performed to probe the recombination mechanisms in these OSCs [33] , [34] . 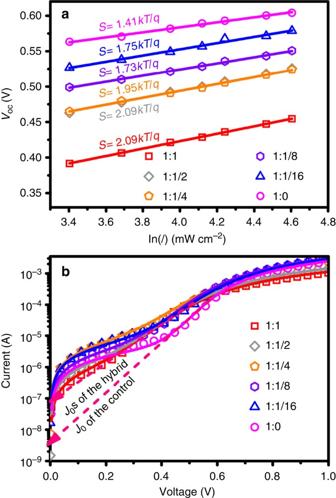Figure 5: Photovoltaic characteristics of hybrid plasmonic OSCs. (a) Intensity-dependent open-circuit voltage measurement and (b) dark current forward bias curve of the AgNPs-P3HT:PCBM and P3HT:PCBM OSCs. Solid lines are the fitted curves. The intercept of the dashed lines with the dark current axis yield the reverse saturation current in these OSCs. Figure 5a shows the V OC versus ln( I ) (where I is the light intensity) for devices with different AgNPs concentration. The slope S = nkT / q , where n is the ideality factor under illumination, k is the Boltzmann constant, T is the temperature and q is the elementary charge, is dependent on the recombination processes in OSCs [35] . In organic systems where first-order trap-assisted recombination is present and competes with Langevin recombination kinetics, intensity-dependent V OC measurements would yield an ideality factor in the range of 1≤ n ≤2. The slope S and other variables from the linear fits of the plots in Fig. 5a are listed in Supplementary Table S1 . S increases from 1.41 kT / q for the control cell to 2.09 kT / q for the hybrid plasmonic cell with the highest AgNPs concentration—clear evidence of increased trap states and increased first-order trap-assisted recombination with increasing AgNPs concentration. In the control cells, at the interface of P3HT:PCBM, traps originating from the defect sites during fabrication, and the intrinsic tail states below the transporting level may contribute to the trap-assisted recombination processes [22] , [27] . At relatively higher concentrations of AgNPs (that is, P3HT:AgNPs ratio >1:1/4), the trap-assisted recombination dominates the kinetics and therefore n approaches 2. Figure 5: Photovoltaic characteristics of hybrid plasmonic OSCs. ( a ) Intensity-dependent open-circuit voltage measurement and ( b ) dark current forward bias curve of the AgNPs-P3HT:PCBM and P3HT:PCBM OSCs. Solid lines are the fitted curves. The intercept of the dashed lines with the dark current axis yield the reverse saturation current in these OSCs. Full size image Dark current analysis To gain a complete picture of the loss mechanisms, dark current analysis measurements were also performed. The dark forward bias characteristics of an OSC are highly dependent on the transport and recombination processes. The common diode equation with the presence of a series resistance R S and a parallel shunt resistance R SH is expressed as: , where n dark is the dark ideality factor, J 0 is reverse saturation current density while k , T and q are the Boltzmann constant, temperature and elementary charge, respectively. Table 3 lists the fitted dark current parameters under forward bias (see Fig. 5b ). J 0 increases by ~2 orders—from 3.32 × 10 −6 to 4.22 × 10 −4 mA cm −2 . Furthermore, n dark increases gradually from 1.66 in the control cells to 2.34 in the cells with the highest Ag concentration—a trend consistent with n (under illumination) in the V OC measurements. It had been shown that the non-ideality of the dark characteristics is dependent on the deeply trapped carriers in the dominant charge transport component of the donor–acceptor blend [35] , [36] . The presence of a high degree of energetic disorder in the density of state (that is, broad trap distribution, deep traps, and so on) of the dominant charge transport phase can result in large ideality factors under dark forward bias. With this understanding, we interpret the increase of n dark (from 1.66 to 2.34) arises from an increase in the energetic disorder stemming from the presence of AgNP-induced subgap traps. Any trap in the charge hopping path would increase the energetic disorder and degrade the charge transport in the film, resulting in a poor dark current injection efficiency. Table 3 Dark current parameters of AgNPs-P3HT:PCBM and P3HT:PCBM OSCs. Full size table Last, in a bid to recreate conditions where AgNP-incorporated devices show improved performance [8] , [9] , we fabricated a set of devices where the P3HT:PCBM films were pre-annealed before Al electrode evaporation. Although the power conversion efficiency of these solar cells were much lower (1.3% versus 3.1% for the optimized devices used in the TAS studies), the performance can be improved with an appropriate amount of AgNPs ( Supplementary Fig. S5 and Supplementary Table S2 ). In such unoptimized devices (with poor carrier mobilities [10] , non-ohmic contact [8] , and so on), the addition of ligand-capped metallic NPs may induce favourable morphology changes, or help improve charge carrier injection between the organic phase and the electrode, thereby improving the performance from factors other than plasmonic effects. These improvements in unoptimized devices could outweigh electron losses through recombination induced by AgNP addition. This could explain the contradictory results presented in previous reports. Plasmonic OSCs provide a viable and highly promising approach for breaking the 10% efficiency barrier of single junction OSCs. Embedding metallic NPs within the active layer offers a highly convenient approach for integrating plasmonic entities in OSCs, where effects like the strong confinement field of localized surface plasmon resonances and enhanced light scattering can be exploited. With intimate proximity to the active layer, these effects can be greatly enhanced. However, the effectiveness of this approach on increasing the efficiencies of OSCs is convoluted by a complex interplay of competing effects. Nonetheless, all these issues may be resolvable through a prudent choice of the constituents and careful optimization of the device. From the analysis of our experimental results and careful comparison with the literature reports [8] , [9] , [10] , [11] , [12] , [13] , we can identify several key factors/considerations for the design of hybrid plasmonic OSCs. The first important factor is the location of plasmonic NPs within the OSC. Given that the plasmonic effects are strongly distance dependent, the incorporation of NPs within the active layer of the OSC would yield the best optical enhancements [3] , [8] , [37] . As concluded from charge dynamic measurements, the existence of these foreign entities introduces traps either through the ligands or the NPs. Although optical enhancement is achieved, these NPs can detrimentally affect the exciton [4] , [6] , [12] , and polaron lifetimes [13] . Thus, as a practical compromise, the plasmonic absorbers would have to be embedded in the charge transport layers (that is, PEDOT:PSS, ZnO, TiO 2 , and so on), as close as possible to the photoactive layers. NP size is another important factor. For good overlap with the optical absorption of the active layer, careful choice of the metal and NP size is required. For best light-scattering effects, the NP size should be of an intermediate size (that is, around 30–60 nm) (ref. 8 ). Although it is generally believed that smaller NPs (<20 nm) can function as subwavelength antennas to couple the enhanced near field to active layer [37] , these smaller NPs have weak light scattering and possess a higher surface-to-volume ratio that can also result in more charge carrier trapping sites. On the other hand, use of NPs that are too big (>60 nm) may bring about deleterious effects of strong metallic absorption; disruption of the BHJ morphology; and shunting problems. In these cases, although plasmonic absorption-induced enhancements may be present, it would be overwhelmed by the above-mentioned concomitant effects. The choice of the capping ligands/outer shells also has an important role, as they can affect the charge transport and morphology of the OSC. They should enable uniform dispersion within the embedding layer, eliminating aggregation of the NPs and disruption of the OSC morphology [12] , [13] , [38] . When embedding the NPs within the active layer, too thin an outer ligand/shell may result in losses via charge/energy transfer between organic materials and the metallic nanostructure [12] . When embedding the NPs within the charge transport layers, poorly capped NPs could still act as charge trapping sites. A combination of an insulating outer shell (for example, SiO 2 ) with an additional organic capping layer (for dispersion) may be able to eliminate such problems. This should be an active area of investigation. To elucidate the true plasmonic contributions in OSCs, a congruence of both transient optical spectroscopies and electrical techniques is of paramount importance. The plasmonic enhancements have to be evaluated in well-optimized devices for further progress in plasmonic OSCs and for true breakthroughs to be made. Elimination of plasmonic NP-induced traps is the limiting factor for attaining high efficiency plasmonic OSCs. In conclusion, ultrafast optical spectroscopy complemented with electrical measurements provides an unambiguous means to probe the charge dynamics and loss mechanisms in organic-ligand-encapsulated AgNPs hybrid plasmonic OSCs. Although an initial increase of exciton generation in these hybrid plasmonic OSCs was observed (with exciton dynamics comparable to that of the control samples), it was found that the high trapping rate of the generated polarons limits the amount of free carriers in the hybrid systems. The carrier dynamics were investigated over the temporal regimes spanning that of generation, recombination, transport and extraction (that is, over 7 orders of magnitude from 100 fs to 5 μs). The AgNPs promote trap-assisted recombination and degrade the performance of the hybrid plasmonic OSCs, as validated by extensive electrical measurements. AgNPs synthesis and characterization The AgNPs were synthesized using a recipe found in the literature [14] —through the reduction of AgNO 3 by oleylamine in refluxing DCB (boiling point: 181 o C). Briefly, 12 mg AgNO 3 (Sigma-Aldrich) was dissolved in 500 μl oleylamine (70%, Sigma-Aldrich) and then rapidly injected into 10 ml refluxing DCB. After 8 h, the reaction was completed. To remove the excessive oleylamine and byproducts, the production solution was added with 30 ml methanol, following by 20-min centrifugation at 4,000 r.p.m. and then redispersed in 10 ml DCB. The above process was repeated three times and the final dry precipitate was dispersed in 10 ml DCB for further use. Device fabrication and electrical characterization Clean patterned indium tin oxide glass was sequentially sonicated in deionized water, acetone and IPA for 15 min each and then cleaned with oxygen plasma. After that, 30 nm PEDOT:PSS was spin coated above the indium tin oxide and then baked at 140 o C in nitrogen atmosphere for 10 min. A 100-nm-thick BHJ layer was subsequently spin coated on top of the PEDOT:PSS layer. The concentration of the P3HT:PCBM used is 10 mg ml −1 :8 mg ml −1 . For the hybrid blends, different ratio of AgNPs in DCB were mixed with the P3HT:PCBM and were spun at 700 r.p.m. for 2 min. The maximum weight ratio of AgNPs:P3HT used is <~3.8%. For better annotation, we had used volume ratio of P3HT:AgNPs (that is, 1:1, 1:1/2, 1:1/4, 1:/1/8, 1:1/16, 1:0) to denote high-to-low AgNPs concentrations in our report. A 100-nm Al metal cathode was evaporated above the BHJ layer and the devices were then baked at 150 o C for 20 min before measurement. Effective area of each cell was 0.071 cm 2 . The current–voltage ( I – V ) characteristics of the devices under illumination and in the dark were recorded with a HP 4155 semiconductor analyser. The cells were illuminated by an Air Mass 1.5 Global (AM 1.5 G) solar simulator (San-Ei XES-300, AAA rating) with an irradiation intensity of 1,000 W m −2 . The performance was averaged over 5–10 cells. The light intensity of the solar simulator was calibrated using a solarimeter with a reference silicon solar cell certified by the National Renewable Energy Lab. The IPCE spectra were recorded using a Merlin radiometry system, where the light source was a 150-W Newport-Oriel Xenon lamp, spectrally resolved using a Cornerstone 260 ¼ m monochromator and chopped at 80 Hz by an optical chopper. The light power-density was calibrated with a Hamamatsu silicon photodiode. All the device tests were performed in an inert nitrogen atmosphere. Optical measurements fs-TAS was performed in a non-degenerate pump-probe configuration. The pump pulses (500 nm) were generated from an optical parametric amplifier (Light Conversion TOPAS) that was pumped by a 1-kHz regenerative amplifier (Coherent Legend; center wavelength: 800 nm; pulse width: 150 fs; power: 1 mJ per pulse), which was in turn seeded by an 80 MHz Coherent Vitesse oscillator. The probe beam was a white light continuum ranging from 450 nm to 1,200 nm generated from a sapphire plate using 800-nm femtosecond pulses. Pump-induced probe transmittance change (relative DT Δ T/T ) was monitored using either a monochromator/PMT configuration (for visible probe range) or a IR-monochromator/InGaAs photodetector configuration (for NIR probe range). The excitation intensity was kept to a minimal of ~6 μJ cm −2 to minimize higher order effects. fs-TAS was performed over a spectral range of 520–1,200 nm and a temporal range from 0 ps to 2 ns to probe the carrier and quasi-particle dynamics in the hybrid plasmonic OSC. ns-TAS was performed using an Applied Photophysics LKS.60 Nanosecond Laser Flash Photolysis Spectrometer with 500-nm excitation pulses generated from a seed Nd:YAG, Q-switched laser (532 nm, 7 ns pulse width), and the probe was a 150-W Xe lamp aligned normal to the excitation source. Each time-resolved trace was acquired by averaging 50 laser shots at a repetition rate of 1 Hz. The typical laser pump fluence used is ~60 μJ cm −2 . The data were collected in transmission geometry with the sample positioned at 45 o with respect to both the excitation source and probe light. TRPL measurements were performed using excitation pulses from the same femtosecond laser system described above. Typically, the samples were photoexcited with a pump fluence of 1.5 μJ cm −2 , and the TRPL signals were collected in a conventional backscattering geometry. The luminescence signal was dispersed by a DK240 1/4-m monochromator with 300 g mm −1 grating, and the temporal evolution of the PL was resolved by an Optronis Optoscope streak camera system, which has an ultimate temporal resolution of ~10 ps when operated at the shortest time window of 330 ps. AgNPs were characterized by transmission electron microscopy (JEM-2010FEF, 200 kV). Steady-state absorption spectra were collected using a Shimadzu UV-3600 UV-VIS-NIR spectrophotometer. How to cite this article: Wu, B. et al. Uncovering loss mechanisms in silver nanoparticle-blended plasmonic organic solar cells. Nat. Commun. 4:2004 doi: 10.1038/ncomms3004 (2013).